Excitonic effects from geometric order and disorder explain broadband optical absorption in eumelanin Eumelanin is a ubiquitous biological pigment, and the origin of its broadband absorption spectrum has long been a topic of scientific debate. Here, we report a first-principles computational investigation to explain its broadband absorption feature. These computations are complemented by experimental results showing a broadening of the absorption spectra of dopamine solutions upon their oxidation. We consider a variety of eumelanin molecular structures supported by experiments or theoretical studies, and calculate the absorption spectra with proper account of the excitonic couplings based on the Frenkel exciton model. The interplay of geometric order and disorder of eumelanin aggregate structures broadens the absorption spectrum and gives rise to a relative enhancement of absorption intensity at the higher-energy end, proportional to the cube of absorption energy. These findings show that the geometric disorder model is as able as the chemical disorder model, and complements this model, to describe the optical properties of eumelanin. Melanin, from the Greek melanos, meaning black color, is a ubiquitous biological pigment. Eumelanin is the most common biological melanin and is responsible for multiple critical functions in living organisms. In humans, eumelanin is the primary determinant of the color of skin, hair and eyes. Besides its pigmentation, eumelanin is also an efficient photoprotective pigment. The broadband absorption spectrum of eumelanin [1] , [2] , [3] , [4] is a result of biological evolution for protecting living organisms from intense sunlight [5] , [6] . Any gaps in the spectrum would leave living organisms vulnerable to these specific wavelengths of sunlight. It has been known that UVA and UVB radiations are major environmental factors that influence the functions and survival of many cell types. Eumelanin is able to dissipate approximately 90% of the UV energy as heat in a nanosecond or even faster time scale [1] , [7] . In addition, studies have demonstrated that visible light can also induce cellular dysfunction and cell death, especially the blue region (400–500 nm), since it has relatively high energies and longer penetration depth [8] . The spectrum of eumelanin has to be monotonically increasing toward the higher-energy end so as to provide an efficient photoprotective function. In order to synthesize biomimetic materials with similar optical properties as eumelanin for industrial or medical applications, a thorough understanding of the intrinsic structural factors and precise mechanisms that give rise to the broadband absorption feature is critical. However, despite significant experimental and theoretical effort over the past several decades, the origin of the broadband absorption spectrum is still a topic of scientific debate, and how the molecular and aggregate structures of eumelanin relate to its overall optical properties is not well understood [9] , [10] . The chemical disorder model is a widely accepted model to explain the broadband absorption spectrum of eumelanin [3] , [11] , [12] . Accordingly, eumelanin consists of many chemically distinct species and its broadband absorption spectrum is a result of averaging over the spectra of these species. The sharp peaks due to 5,6-dihydroxyindole (DHI) and its oligomers could be eliminated after this process [3] , [11] , [12] , [13] , [14] , [15] , [16] . Even though the chemical disorder model combined with the superposition principle are able to reproduce broadband absorption spectra, they are, however, still insufficient to provide a full explanation of the optical properties of eumelanin. First, experiments have confirmed that eumelanin is made of stacked oligomers with an interlayer distance 3–4 Å (refs 17 , 18 ). It is expected that when molecules are brought close to this extent, the electron density and spectrum will change. Studies have shown that the interactions among eumelanin protomolecules are strong enough to affect the spectrum significantly, where the superposition principle clearly does not hold [14] . Second, the molecular structures of eumelanin are still poorly understood, and so are the ratios of distinct species. It is less convincing that overfitting does not occur when averaging over chemical inhomogeneity. Third, the chemical disorder model requires many distinct species of eumelanin protomolecules to reproduce broadband absorption spectra. However, these families of molecules have not been shown to reproduce other important properties of eumelanin, such as its mechanical properties and aggregate structures. Last but not least, the chemical disorder model is unable to explain why the spectrum of eumelanin is monotonically increasing toward the higher-energy end, which is one of the most important spectroscopic features of eumelanin. There have been several attempts to calculate the spectra of eumelanin. However, due to computational limitations, the system sizes were limited to no more than three molecules [11] , [13] , [14] , [15] , [16] , [19] , [20] . Such a setup is unable to capture the full picture of the optical properties of eumelanin since it neglects the geometric disorder characteristic. It is necessary to go beyond these studies and to consider more realistic systems, which introduce the effect of geometric disorder through ensemble sampling. Although the molecular structures of eumelanin are still undefined, previous experimental reports provided important constraints and suggestions for choosing the molecular models. X-ray diffraction studies [21] , [22] and scanning tunneling microscopy measurements [23] , [24] , [25] showed that the size of eumelanin protomolecules is around 15–20 Å, which suggested that the tetramers and pentamers formed by covalently bonded DHIs are the most possible molecular structures of eumelanin. Matrix-assisted laser desorption/ionization mass spectrometry studies [26] , [27] , [28] , [29] , [30] , [31] showed that the mass of eumelanin protomolecules is within or below ~600–1,200 amu, and large polymeric structures are not observed, with the exception of the data reported in a recent report [32] . Hence, most of the investigations performed by mass spectrometry supported that the tetramers and pentamers constitute the majority of eumelanin, while slightly larger structures, such as the hexamers and octamers, are also possible. We note that Dreyer et al. [33] recently proposed a new molecular model for poly(dopamine) and eumelanin, based on a variety of solid state spectroscopic and crystallographic techniques. Their study suggested that eumelanin are supramolecular aggregates of monomers. Here, we consider a variety of eumelanin molecular structures supported by experiments or theoretical studies. These models include a monomeric model proposed by Dreyer et al. [33] , tetrameric model proposed by Kaxiras et al. [16] , [19] , as well as pentameric and octameric models proposed by Cheng et al. [21] , [22] , which cover a broad range of the most possible molecular structures of eumelanin. In addition, other models proposed and experimentally validated by Panzella et al. [34] and Arzillo et al. [35] are also considered. The spectra of small-scale systems made of these models are obtained through conventional quantum chemical calculations, and the Frenkel exciton model is invoked to calculate the spectra of large-scale systems. It is found, as an entirely new result, packing disorder of a single species of DHI oligomer is as successful as and even better than the chemical disorder model. We find that the increase in oscillator strength toward the higher-energy end of the spectrum as a result of the excitonic couplings among eumelanin protomolecules. In addition, the absorption spectra of dopamine solution taken as functions of time in oxidative conditions are consistent with the results of our simulations. Absorption spectra of small-scale systems The molecular structures of eumelanin considered in this work have distinct optical characteristics in the gas phase, in line with the chemical disorder model. The individual molecular structures are shown in Fig. 1a–d . We begin our investigation from small-scale systems. The geometry of a single molecule of each model in the gas phase is optimized using density functional theory (DFT) calculations (see Methods Section for details). However, it is computationally demanding to perform DFT on the systems with more than one molecule, and the proper account of van der Waals interactions in DFT is an open subject of study. We perform molecular dynamics (MD) simulations to find the equilibrium structures of the systems that contain more than one molecule. The equilibrium structures of the small-scale systems are shown in Fig. 1e–l . On the basis of these structures, we use ZINDO/S method to calculate the spectra of the small-scale systems and the results are shown in Fig. 2 . Several sharp peaks in the spectra are observed, which are the expected results for small organic molecules. These results clearly show that the spectra of eumelanin protomolecules change as a function of aggregate size. We also find similar results for different molecular models (see Supplementary Discussion and Supplementary Figs 1 and 2 for details) and different redox states (see Supplementary Discussion and Supplementary Figs 3 and 4 for details). These results indicate the inadequacy of calculating the spectrum of eumelanin using the superposition principle since it simply ignores the excitonic couplings among the eumelanin chromophores. 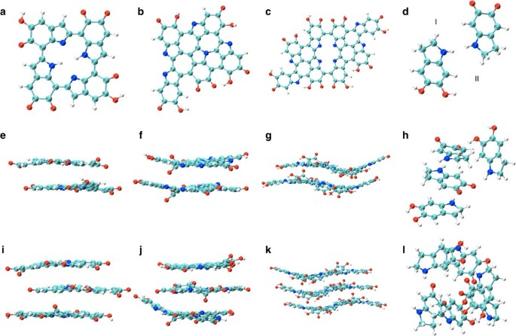Figure 1: Molecular models and equilibrium structures of small-scale system. (a) Tetrameric model proposed by Kaxiraset al.16,19(b) Pentameric model and (c) octameric models proposed by Chenget al.21,22(d) Monomeric model proposed by Dreyeret al.33There are two monomers in the monomeric model, and we call them M1 and M2 in this work. Two-layer stacked structure of the (e) tetrameric model, (f) pentameric model and (g) octameric model, respectively. (h) Two-set (two M1 monomers and two M2 monomers) stacked structure of the monomeric model. Three-layer stacked structure of the (i) tetrameric model, (j) pentameric model and (k) octameric model, respectively. (l) Three-set (three M1 monomers and three M2 monomers) stacked structure of the monomeric model. These equilibrium structures are obtained from the MD simulations with the NVT ensemble at a constant temperature of 300 K for 2.0 ns. Figure 1: Molecular models and equilibrium structures of small-scale system. ( a ) Tetrameric model proposed by Kaxiras et al. [16] , [19] ( b ) Pentameric model and ( c ) octameric models proposed by Cheng et al. [21] , [22] ( d ) Monomeric model proposed by Dreyer et al. [33] There are two monomers in the monomeric model, and we call them M1 and M2 in this work. Two-layer stacked structure of the ( e ) tetrameric model, ( f ) pentameric model and ( g ) octameric model, respectively. ( h ) Two-set (two M1 monomers and two M2 monomers) stacked structure of the monomeric model. Three-layer stacked structure of the ( i ) tetrameric model, ( j ) pentameric model and ( k ) octameric model, respectively. ( l ) Three-set (three M1 monomers and three M2 monomers) stacked structure of the monomeric model. These equilibrium structures are obtained from the MD simulations with the NVT ensemble at a constant temperature of 300 K for 2.0 ns. 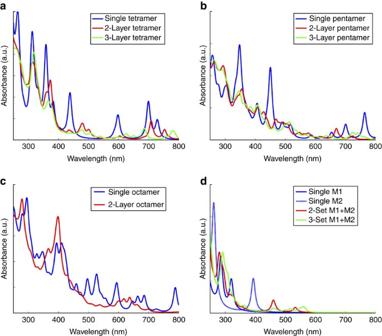Figure 2: Absorption spectra of small-scale systems. The respective spectra are calculated directly with ZINDO/S method. Due to the proximity of the stacked eumelanin protomolecules, it can be seen that the significant excitonic interactions qualitatively change the landscape of the spectra. Full size image Figure 2: Absorption spectra of small-scale systems. The respective spectra are calculated directly with ZINDO/S method. Due to the proximity of the stacked eumelanin protomolecules, it can be seen that the significant excitonic interactions qualitatively change the landscape of the spectra. Full size image Absorption spectra of large-scale systems The snapshots of the large-scale systems after the MD simulations (see Methods Section for details) are shown in Fig. 3 . The snapshots of the oligomeric models (namely the tetrameric, pentameric and octameric models) reveal simulated aggregate structures, which are similar to those observed experimentally [17] , [18] . However, we cannot find similar aggregate structures in the snapshot of the monomeric model. In addition to the aggregate structures, the oligomeric models are also able to reproduce the mechanical properties of eumelanin including the mass density and Young’s modulus in good agreement with the experimental measurements [36] , [37] , [38] , [39] (see Supplementary Discussion and Supplementary Fig. 5 for details). In accordance with our previous work [17] , the aggregate size (secondary structure) distribution of eumelanin extends to a dozen of eumelanin protomolecules ( Supplementary Fig. 6 ). In the MD simulations, the eumelanin protomolecules tend to adopt random-like orientations ( Supplementary Fig. 7 ) and stack together to form secondary structures with different aggregate sizes. In the large-scale systems, there are only 29 tetramers (that is, 4.0%), 66 pentamers (9.3%) and 129 octamers (17.7%) among 729, not forming secondary structures. For the monomeric model, there are 437 monomers (30%) among 1,458 (729-set) not forming secondary structures. These results imply that the random-like arrangement (entropic contribution) with stacked eumelanin protomolecules (enthalpic contribution) is thermodynamically more favorable than ordered arrangements. The simulated aggregate structures with geometric disorder characteristic are actually in good agreement with experimental observations [17] , [18] . 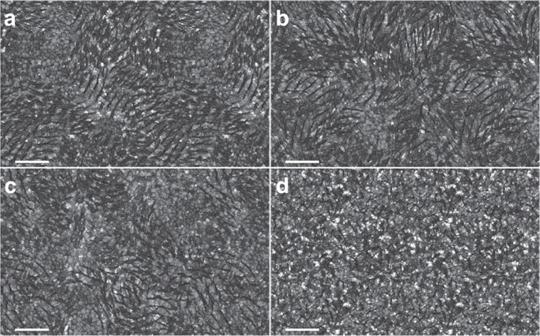Figure 3: Snapshots of large-scale systems obtained from MD simulation. The aggregate structures of the (a) tetrameric, (b) pentameric, (c) octameric and (d) monomeric model, respectively. The snapshots of the oligomeric models (namely the tetrameric, pentameric and octameric models) reveal simulated aggregate structures that are similar to those observed experimentally17,18. However, we cannot find similar aggregate structures in the snapshot of the monomeric model. Scale bar, 2 nm. Figure 3: Snapshots of large-scale systems obtained from MD simulation. The aggregate structures of the ( a ) tetrameric, ( b ) pentameric, ( c ) octameric and ( d ) monomeric model, respectively. The snapshots of the oligomeric models (namely the tetrameric, pentameric and octameric models) reveal simulated aggregate structures that are similar to those observed experimentally [17] , [18] . However, we cannot find similar aggregate structures in the snapshot of the monomeric model. Scale bar, 2 nm. Full size image One expects that the spectra will continue to change as a function of aggregate size. However, the calculations of the spectra of the systems that contain more than few eumelanin protomolecules are beyond the capability of quantum chemical methods. We calculate the spectra of the large-scale systems obtained from the MD simulations with proper account of the excitonic couplings based on the Frenkel exciton model [40] . The basis of the Frenkel exciton model is spanned by the singly excited states of the constituent eumelanin protomolecules in the gas phase, calculated with ZINDO/S method. In addition, for an accurate estimation of the excitonic interactions, we adopt the atomic transition charge distribution method instead of the more popular point dipole method. This is necessary since the interlayer distance observed in the MD simulations is approximately 3–4 Å, even smaller than the typical dimension of the eumelanin protomolecules. The point dipole method is known to give failing estimations of the excitonic couplings to the extent of an order of magnitude in such circumstances [41] , [42] , [43] . We show that the Frenkel exciton model is accurate in calculating the spectra of eumelanin protomolecules since it is able to provide similar results as those obtained using ZINDO/S method (see Supplementary Discussion and Supplementary Fig. 8 for details). The spectra of the large-scale systems calculated using the Frenkel exciton model are shown in Fig. 4 . It appears that the simulated spectra of the aggregate structures are drastically different from those of the oligomers in the gas phase. For the oligomeric models ( Fig. 4a–c ), the simulated spectra appear to have similar characteristics as the experimental results [1] , [2] , [3] , [4] , namely being smooth and monotonically increasing toward the higher-energy end. However, the spectra of the monomeric model ( Fig. 4d ) show that the monomers actually cannot absorb visible light, which is in marked contrast with the experimental spectra of eumelanin suspensions [9] , [10] , [11] . In addition, the spectra of the systems containing 27 oligomers (or 54 monomers) are similar to those of containing 729 oligomers (or 1,458 monomers). This suggests that the large-scale systems in this work are large enough to capture the full picture of the optical properties of eumelanin. In other words, the delocalization length of the exciton is much smaller than the box size. This result holds not only for the possibly hypothetical planar tetrameric model proposed by Kaxiras et al. [16] , [19] , and for the planar pentameric and octameric models proposed by Cheng et al. [21] , [22] , but also for the non-planar oligomers (see Supplementary Discussion and Supplementary Figs 1 and 2 for details) whose presence in solution has been demonstrated experimentally [34] , [35] . 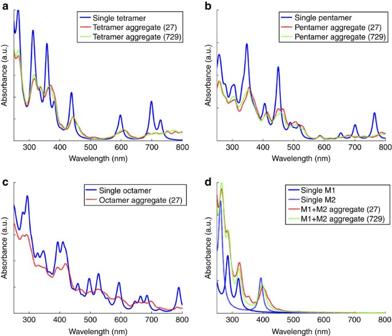Figure 4: Absorption spectra of large-scale systems. In line with the discussion inFig. 2, here the spectra of the corresponding large-scale systems are shown. While in this case full-scale quantum chemistry calculation is not feasible, we account for the excitonic interactions through the Frenkel exciton model with the atomic transition charge distribution method. Figure 4: Absorption spectra of large-scale systems. In line with the discussion in Fig. 2 , here the spectra of the corresponding large-scale systems are shown. While in this case full-scale quantum chemistry calculation is not feasible, we account for the excitonic interactions through the Frenkel exciton model with the atomic transition charge distribution method. Full size image Absorption spectra of dopamine solutions during its oxidation The simulated spectra of eumelanin share many common features with the experimental ones ( Fig. 5a ). Specifically, after short oxidation times of dopamine solutions (2 mg ml −1 in the presence of Tris buffer and using O 2 from the air as an oxidant, see Methods Section for details), a small peak appears at λ max =724 nm, absent from the dopamine solutions, in the absorption spectra of the diluted dopamine–eumelanin solutions. This peak position is close to that predicted for the tetramers and pentamers but markedly different from that of the octamers. This could imply that such porphyrin like structures as those corresponding to the tetramers ( Fig. 1a ) appear indeed during the formation of dopamine–eumelanin in solution. A definitive proof for the presence of such molecules is nevertheless required. Unfortunately, NMR spectroscopy is not sensitive enough to detect such molecules at such low concentrations. When the reaction time increases, the relative contribution of the absorption peak at 724 nm decreases in favor of a more broadband absorption, characteristic of eumelanin ( Fig. 5b ). This is exemplified by a marked decrease of the absorbance ratio at 724 nm and at 500 nm, a wavelength at which eumelanin absorbs but at which only the octameric model used in the simulations absorbs significantly ( Fig. 4c ). Simultaneously, the absorbance ratio at 420 nm and at 500 nm increases with the reaction time, showing that the absorbance markedly increases in the higher-energy end of the spectrum, a well known observation for eumelanin, the finding also predicted in the simulations ( Fig. 4 ). Hence, the time evolution of the experimental spectra is parallel to the evolution of the simulated spectra for which the aggregate size increases reflecting the self-assembly process of eumelanin protomolecules. 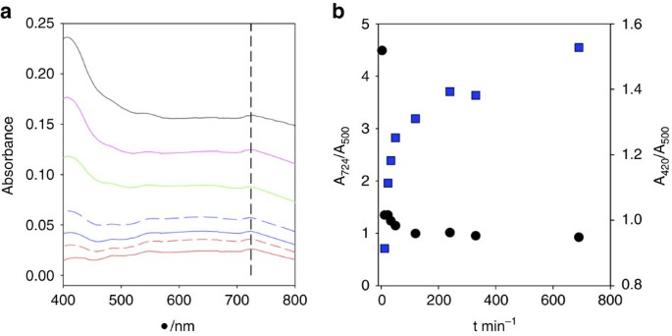Figure 5: Absorption spectra of dopamine solutions during its oxidation. (a) Absorption spectra of dopamine solutions (2 mg ml−1in the presence of 50 mM Tris buffer at pH=8.5 in the presence of oxygen from the air and at 25±1 °C) taken at different times after the dopamine solution was prepared, and diluted by a factor of 6 before spectral characterization: 12 min (red line), 24 min (red dashed line), 34 min (blue line), 50 min (blue dashed line), 2 h (green line), 4 h (purple line), 5 h and 30 min (black line). For clarity, the absorption spectra measured at longer reaction times are not displayed. The dashed vertical line indicates the absorption band at 724 nm. (b) Absorbance ratios, A724/A500(black circles, left hand vertical scale) and A420/A500(blue squares, right hand vertical scale) as a function of the reaction time. The absorbance values were taken from the spectra displayed in parta. Figure 5: Absorption spectra of dopamine solutions during its oxidation. ( a ) Absorption spectra of dopamine solutions (2 mg ml −1 in the presence of 50 mM Tris buffer at pH=8.5 in the presence of oxygen from the air and at 25±1 °C) taken at different times after the dopamine solution was prepared, and diluted by a factor of 6 before spectral characterization: 12 min (red line), 24 min (red dashed line), 34 min (blue line), 50 min (blue dashed line), 2 h (green line), 4 h (purple line), 5 h and 30 min (black line). For clarity, the absorption spectra measured at longer reaction times are not displayed. The dashed vertical line indicates the absorption band at 724 nm. ( b ) Absorbance ratios, A 724 /A 500 (black circles, left hand vertical scale) and A 420 /A 500 (blue squares, right hand vertical scale) as a function of the reaction time. The absorbance values were taken from the spectra displayed in part a . Full size image Spectral broadening from random excitonic interactions Intriguingly, the peaks at the lower-energy end of the spectra are broadened and lowered substantially compared with those at the higher-energy end. Two main factors contribute to this observation. First, the excitonic interactions among the stacked eumelanin protomolecules are enhanced due to the short interlayer distance 3–4 Å. This essentially grants the excitons extended radii over a number of neighboring molecules. The energies of the excitons are then redistributed within the range of approximately , where is the average nearest neighbor coupling strength, centered at the gas phase peak locations [44] . Second, on close inspection of the microscopic details of molecular arrangement obtained through the MD simulations, no correlation of molecular orientations within individual secondary structures is observed. In other words, the self-assembly mechanism of eumelanin protomolecules is characterized only through reducing intermolecular separations and the alignment of molecular planes, whereas molecules are allowed to freely rotate with respect to the axis of aggregations. This is due to both the isotropy and weakness of the intermolecular forces compared with the kinetic energy at physiological temperatures. Consequently, the oscillator strength is redistributed more or less evenly within the range as mentioned above. This is in sharp contrast to the phenomenon of exchange narrowing typically observed in molecular aggregate systems having well-defined geometries, especially with definite orientation order [45] . Generically, we observe that the gas-phase absorption peaks of the eumelanin protomolecules are redistributed when they randomly stack together and are allowed to interact via excitons. Moreover, this redistribution is carried out in such a way that ones with lower transition energies are spread to a larger extent than others. Put differently, the low energy transitions are attenuated compared with the high energy ones on the formation of secondary structures. This results in the rather featureless spectrum in which the absorbance increases toward the higher-energy end in a monotonic manner, in agreement with the experimental findings [9] , [10] , [11] . A simple explanation can be given to rationalize this observation: using the tetrameric model as an example, let us consider a simpler situation, where we retain only two absorption peaks of individual molecule, one located at 358 nm and another at 699 nm with similar oscillator strengths (64.7 Debye and 61.3 Debye [2] from ZINDO/S method, respectively), and perform the Frenkel exciton model calculation with the same aggregate structure (729 tetramers shown in Fig. 3a ). These two absorption peaks are located at the two extremities of the visible spectrum. The simulated spectra of this simplified system are shown in Fig. 6a,b . As indicated in the figure, we first note that there is no noticeable intensity borrowing effect [46] between the two energetically well-separated bands, since the ratio between the integrated intensities are the same for the gas phase and aggregate structure. In frequency space ( Fig. 6a ), the bandwidth of these two bands is roughly the same (6.0 × 10 3 cm −1 for the lower-energy band and 7.5 × 10 3 cm −1 for the higher-energy band). However, when plotted in wavelength space ( Fig. 6b ), the bandwidth of these two bands appears to be drastically changed relative to each other: the higher-energy band is much narrower than the lower-energy band. 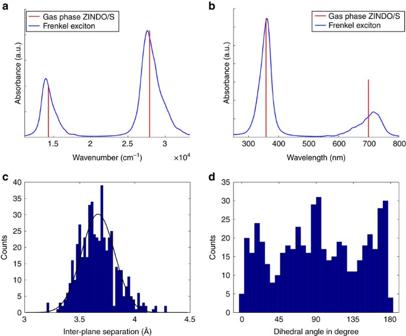Figure 6: Absorption spectra of simplified system and in-depth analysis of MD simulation trajectory. The panels depict a comparison of the same absorption spectrum in (a) frequency and (b) wavelength space, calculated with the same aggregate structure (729 tetramers shown inFig. 3a) but using only two transitions (Ek=2.79 × 104,1.43 × 104(cm−1) or (λk=358,699 (nm) and oscillator strengths (fk=64.7,61.3(Debye2)) per molecule. The red sticks correspond to the result from ZINDO/S method for the gas phase, and the blue line represents the result of the Frenkel exciton calculation for the aggregate structure. (c) The distribution of plane-to-plane distances. The mean value is 3.67 Å with a s.d. of 0.15 Å, when fitted to a Gaussian distribution. (d) The distribution of dihedral angles among the adjacent molecules. The result indicates that there is no favorite rotational configuration of the stacked eumelanin protomolecules. Figure 6: Absorption spectra of simplified system and in-depth analysis of MD simulation trajectory. The panels depict a comparison of the same absorption spectrum in ( a ) frequency and ( b ) wavelength space, calculated with the same aggregate structure (729 tetramers shown in Fig. 3a ) but using only two transitions ( E k =2.79 × 10 4 ,1.43 × 10 4 (cm −1 ) or ( λ k =358,699 (nm) and oscillator strengths ( f k =64.7,61.3( Debye 2 )) per molecule. The red sticks correspond to the result from ZINDO/S method for the gas phase, and the blue line represents the result of the Frenkel exciton calculation for the aggregate structure. ( c ) The distribution of plane-to-plane distances. The mean value is 3.67 Å with a s.d. of 0.15 Å, when fitted to a Gaussian distribution. ( d ) The distribution of dihedral angles among the adjacent molecules. The result indicates that there is no favorite rotational configuration of the stacked eumelanin protomolecules. Full size image The above observation is rationalized as follows. The average excitonic couplings of these two excitations within the single excitation manifold ( ) are similar. Therefore, and as stated previously, the width of the bands is also similar in frequency (energy) space. In other words, the location and the range of the bands can be represented as , where E k is the energy of the k th gas phase absorption peak (in wavenumber) and α is a dimensionless constant. The same expression in wavelength space is where 10 7 is the transformation factor relating wavenumbers and wavelengths. λ k =10 7 / E k is the wavelength of the k th transition in nanometer, and α ′=10 7 · α is the proportionality factor in wavelength space. We truncate the Taylor series to the first order in , which is typically on the order of 10 −1 to 10 −2 in our calculations and is characteristic of molecular aggregates in the visible light region [40] . Note that the bandwidth is now proportional to . In our simplified two-state calculation, this means that the ratio of the width of the two bands is multiplied by a factor of ( E 1 / E 2 ) 2 =3.8, in favor of the band with higher energy. Moreover, due to the sum rule of oscillator strength, this corresponds to a relative increment in the absorption intensity by a factor of 3.8. Another factor comes from the fact that the absorbance is proportional to the product of oscillator strength and transition energy. In typical spectroscopic studies on molecular aggregates, one usually focuses only on the oscillator strength and takes the transition energy as constant. This is, as mentioned, due to the fact that the absorption intensities of molecular aggregates with well-defined geometries are concentrated at the upper or lower band edges, for H- or J- aggregates [47] , respectively. However, in this work, the energy range under discussion is very broad, and the lack of ordered aggregate structures precludes the intensity-concentration effect. Apart from the oscillator strength characteristic of the selected eumelanin protomolecules, there is an additional factor of transition energy contributing to the absorption intensity. The above argument also applies to the general situation where all gas phase transitions (instead of just two) are included. Moreover, this argument is not limited to the systems that consists only one kind of molecular structure, and is also compatible with the chemical disorder model. Geometric order and disorder as seen from statistics To support the above argument, we use the same aggregate structure (729 tetramers shown in Fig. 3a ) as an example and present a more in-depth analysis to the MD simulation trajectory. The statistical analysis on the geometry of adjacent molecules is shown in Fig. 6c,d . In Fig. 6c , we plot the distribution of interlayer distances between adjacent molecules. The definition of intermolecular adjacency is provided in Supplementary Methods and Supplementary Figs 9,10 and 11 . The distribution has a Gaussian form with mean value of 3.67 Å, which correlates well with the experimental observations [17] , [18] . In addition, the distribution of the dihedral angles between adjacent molecules is shown in Fig. 6d . We conclude that there is no favorite rotational configuration of the stacked molecules at physiological temperatures. The above observations, consistent with the experimental findings that there is no crystalline order within eumelanin aggregate structures [17] , [18] , is crucial to our explanation of the broadband absorption feature induced by excitonic couplings. This kind of disorder destroys the intensity-concentrating effect typically observed in molecular (H- or J-) aggregates with rotational ordering. In the rotationally disordered eumelanin aggregate structures, the oscillator strength is scattered across the full range of the band, spanned by the excitonic couplings. From the above analysis, we conclude that the geometric order together with disorder originating from the thermodynamics of the large-scale systems lead to the peculiar characteristics of the optical properties of eumelanin. The geometric order refers to stacking of the planar eumelanin protomolecules with nearest separation in the range of 3–4 Å, whereas the geometric disorder concerns the lack of preference on the rotational degrees of freedom between adjacent molecules, as well as the slipping along the molecular planes. On the one side, the geometric order characteristic gives rise to significant excitonic couplings among eumelanin protomolecules. On the other side, the geometric disorder scatters the absorption intensity over the exciton energy band. To the best of our knowledge, the absorption spectra of eumelanin aggregate structures containing hundreds of eumelanin protomolecules with proper account of the excitonic couplings are calculated for the first time. We show that the inclusion of excitonic interactions among eumelanin protomolecules drastically changes the landscape of the spectrum, which mimics the one obtained experimentally. The interplay of geometric order and disorder characteristics of eumelanin aggregate structures results in significant and random excitonic couplings among the molecules. Consequently, these couplings broaden the spectrum and give rise to a relative enhancement of absorption intensity to the higher-energy end, which is proportional to the cube of the absorption energy. While we do not explicitly include chemical disorder and the spectra are calculated individually for each molecular model, this principle is compatible to the general case including chemical inhomogeneity. We note that several groups have considered the effect of dynamical disorder [48] , [49] , where short-range interactions among nearby molecules affect the molecular geometry dynamically. However, as in the case of chemical (static) disorder model, the excitons are still restricted within one (segment of a) molecule since their interactions are neglected in these studies. As such, the delocalization of excitons over several neighboring eumelanin protomolecules will prove crucial for comprehensive understanding of the broadband absorption feature. This work shows that the excitonic effect can play a decisive role in the interpretation of the broadband absorption spectrum of eumelanin. The significance of the excitonic couplings is strongly suggested by the fact that eumelanin is composed of (a mixture of) conjugated molecules and the short interlayer distance among the stacked eumelanin protomolecules shown in both the MD simulations and experiments. On top of that, we further find that the rotational disorder and slip along molecular planes within individual secondary structures are also key ingredients to the spectroscopic features of eumelanin. Our results confirm the model of heterogeneous aggregation for eumelanin, but in a different way than the previous reports that deal with the simulations of the optical properties of eumelanin based solely on the superposition principle. In these earlier reports, the heterogeneity originated from a chemical point of view since different eumelanin protomolecules were used to calculate the spectra. In contrast, our heterogeneity comes from the fact that the stacked eumelanin protomolecules are in different sizes and randomly oriented, leading to the peculiar excitonic interactions among them. More broadly, we demonstrate that in addition to the exact chemical identity of eumelanin, which differs from one kind of molecules to another, there exists a universal enhancement of absorption intensity to the cube of the absorption energy. Therefore, the overall shape of the eumelanin spectrum, which is broadband and smoothly decaying to the lower-energy end, can be rationalized accordingly. It should be noted that although the chemical disorder model can explain the broadband absorption feature of eumelanin, it is unable to explain why the spectrum of eumelanin is monotonically increasing toward the higher-energy end. In contrast, this work explains both important optical characteristics of eumelanin. The concept uncovered here has implications beyond the specific microscopic models of eumelanin, and provides an important advance in the understanding of the optical properties of other materials with similar chemical and structural characteristics. It may also enable the design of bio-inspired materials with similar optical properties as eumelanin. All-atom modeling and equilibration Full atomistic MD simulations are performed using the large-scale atomic/molecular massively parallel simulator with the consistent valence force field (CVFF). The CVFF is parameterized to reproduce peptide and protein properties and has been supplemented with several parameters for small organic molecules including dopamine [50] . The CVFF is accurate in simulating the eumelanin protomolecules considered in this work since the results calculated using MD simulations with the CVFF are very close to those calculated using DFT (see Supplementary Discussion and Supplementary Fig. 12 , Table 1 and 2 for details). Energy minimization using the conjugate gradient algorithm is performed before the MD simulations. The integration time step is set as 0.5 fs, and the nonbonding interactions (12/6 Lennard–Jones and Coulomb interactions) are computed using a cutoff for neighbor list at 12.0 Å. Periodic boundary conditions are used in the MD simulations. In this work, the large-scale systems contain 27 and 729 oligomers (namely the tetrameric, pentameric and octameric models) or 54 (27-set) and 1,458 (729-set) monomers. The initial distance between the molecules is set to be around 30 Å, to ensure that there are no intermolecular interactions in the initial configuration. After energy minimization, the systems are simulated with the NPT ensemble at a constant temperature of 1,000 K and pressure of 1.013 bar for 2.0 ns, to ensure sufficient exploration on the configurations of the final aggregate structures. The high temperature allows the molecules to reach the most stable configurations much faster than at room temperature (300 K). However, we notice that there might be some vacancies in the systems after the previous NPT ensemble, and these vacancies might remain in the systems for a long time even after we cool down the temperature to 300 K. In order to remove these vacancies, the systems are then simulated with the NPT ensemble at a constant temperature of 300 K and pressure of 10,130 bar for another 2.0 ns. The high pressure compresses the systems and therefore removes these vacancies. Since we are interested in the optical and mechanical properties of eumelanin at room temperature (300 K) and standard atmospheric pressure (1.013 bar), the systems are then simulated with the NPT ensemble at a constant temperature of 300 K and pressure of 1.013 bar for another 2.0 ns. Calculations of absorption spectra The molecular models of eumelanin are first optimized using DFT implemented in ORCA [51] with B3LYP exchange correlation functional and Ahlrichs-VDZ polarized basis set [52] . These optimized structures are then used as the inputs of ZINDO/S method implemented in Gaussian 09 [53] to calculate the spectra in the gas phase. A Lorentzian broadening with FWHM of 7.5 nm has been applied to the raw results in order to generate Fig. 2 . The raw results are used as the inputs of the Frenkel exciton model to calculate the spectra of the large-scale systems. In Fig. 2c , we do not provide the result of the three-layer octamer due to computational limitations (the octameric model contains much more atoms than the other models). In order to include the excitonic effect emerges upon eumelanin aggregations, we adopt the standard Frenkel exciton model [40] . The Frenkel exciton model takes into account only the singly excited manifolds of the molecules of interest, which is appropriate for this work. Here, we ignore both the spectral broadening effects originating from static (inhomogeneous) and dynamical (homogeneous) disorders for simplicity. Taking ħ =1, the Hamiltonian reads where ω m,i is the transition energy of the i th transition of molecule m . Since we consider no chemical disorder throughout the system, we simply set ω m,i = ω i , that is, the transition energies are independent of the site label. | m , i 〉 denotes the state in which the i th electronic transition of the m th molecule is excited, while all other molecules in the system are in their ground state. N M and N S are the size of the aggregate structure and number of monomeric transitions included in the calculation, respectively. Note that the summations over m and n in the second term exclude the case where m = n , in other words, there is no coupling between transitions within the same molecule. J ( m,i;n,j ) specifies the coupling between the i th transition of the m th molecule and the j th transition of the n th molecule. As mentioned before, we adopt the atomic transition charge distribution method [54] , [55] , thus where is the transition electron density between the ground state and i th excited state on the k th atom. r kl is the separation between corresponding atoms, taken from the results of the MD simulations described before. The summations run overall the atoms of molecules m ( M m ) and n ( M n ), and the linear absorption spectrum of the system is obtained by numerically diagonalizing the Hamiltonian. The terms in the parentheses insure that the interaction exists only between different molecules. In this work, we include 48 electronic transitions of the molecules with largest oscillator strengths, that is, N s = 48 . The absorption spectra show no noticeable difference by either increasing the system size ( N m ) or the number of gas phase transitions included ( N s ). A Lorentzian broadening with FWHM of 7.5 nm has been applied to the raw results in order to generate Fig. 4 . In Fig. 4c , we do not provide the result of the large-scale system containing 729 octamers due to computational limitations (the octameric model contains much more atoms than the other models). Absorption spectra of dopamine solutions during its oxidation Dopamine hydrochloride (Sigma Aldrich H8502) was dissolved in 50 mM Tris Buffer (pH=8.50 adjusted with hydrochloric acid) to undergo its oxidation in the presence of O 2 from the air. The dissolution of dopamine defined the beginning of the oxidation kinetics. The dopamine containing solution was vigorously shaken with a magnetic stirrer ( ω =300 r.p.m.) and at ambient temperature, 25±1 °C. At regular time intervals, 500 μl of this solution was removed from the reaction mixture and diluted by a factor of 6 with Tris buffer and its absorption spectrum was immediately measured with a Cary 100 double beam spectrophotometer (Varian) between 400 and 800 nm. The absorption spectra are not displayed at shorter wavelengths because they display a high absorption peak at around 280 nm due to dopamine. However, a non-oxidized dopamine solution does not absorb at all above 320 nm. Hence, the displayed absorption spectra display the spectral contribution of the oxidation products of dopamine. The absorption spectra were measured against Tris buffer taken as a reference. How to cite this article: Chen, C.-T. et al. Excitonic effects from geometric order and disorder explain broadband optical absorption in eumelanin. Nat. Commun. 5:3859 doi: 10.1038/ncomms4859 (2014).